RETRACTED ARTICLE: Pharmacological perturbation of CXCL1 signaling alleviates neuropathogenesis in a model of HEVA71 infection Hand, foot and mouth disease (HFMD) caused by Human Enterovirus A71 (HEVA71) infection is typically a benign infection. However, in minority of cases, children can develop severe neuropathology that culminate in fatality. Approximately 36.9% of HEVA71-related hospitalizations develop neurological complications, of which 10.5% are fatal. Yet, the mechanism by which HEVA71 induces these neurological deficits remain unclear. Here, we show that HEVA71-infected astrocytes release CXCL1 which supports viral replication in neurons by activating the CXCR2 receptor-associated ERK1/2 signaling pathway. Elevated CXCL1 levels correlates with disease severity in a HEVA71-infected mice model. In humans infected with HEVA71, high CXCL1 levels are only present in patients presenting neurological complications. CXCL1 release is specifically triggered by VP4 synthesis in HEVA71-infected astrocytes, which then acts via its receptor CXCR2 to enhance viral replication in neurons. Perturbing CXCL1 signaling or VP4 myristylation strongly attenuates viral replication. Treatment with AZD5069, a CXCL1-specific competitor, improves survival and lessens disease severity in infected animals. Collectively, these results highlight the CXCL1-CXCR2 signaling pathway as a potential target against HFMD neuropathogenesis. Human Enterovirus A71 (HEVA71) is a small, positive-sense, single-stranded RNA virus that was first isolated in 1969 from patients with severe central nervous system diseases [1] . It has since emerged as one of the most important causative agents of hand, foot and mouth disease (HFMD), a serious global public health threat with epidemic outbreaks in the Asia-Pacific regions with high annual disability-adjusted life years (DALYs) [2] , [3] . Despite its severity, there is a paucity of treatments currently available to affected patients [4] . While usually a benign and self-limiting infection, a substantial portion of HEVA71-infected children under 3 years of age continue to develop serious neurological deficits including aseptic meningitis, brain stem encephalitis and poliomyelitis-like acute flaccid paralysis that can culminate in permanent neurological sequelae or even fatality [5] , [6] . Post-mortem studies confirmed the presence of HEVA71 infection in the central nervous system (CNS), particularly in the medulla oblongata and spinal cord, indicating that the neurological complications are linked to viral replication in the CNS [7] , [8] . Dysregulated cytokine production is strongly linked to severe HEVA71 infections with neurological complications [9] . In particular, cytokines modulated by specific HEVA71 proteins are known to be hijacked by the virus to subvert host responses [10] . For example, the 2A protease reduces type I IFN receptor (IFNAR1) expression, preventing interferon (IFN)-facilitated antiviral responses in skeletal muscle cells [11] . Similarly, the 3C protease suppresses mitogen-activated protein kinase (MAPK) signaling to reduce the expression of anti-viral pro-inflammatory cytokines in intestinal epithelial cells [12] . However, the identities of CNS-specific cytokines and the viral proteins directly responsible for modulating their production remains undefined [13] , [14] . There remains a critical knowledge gap surrounding the relationship between these cytokines and their contributions to neurological complications in severe cases and fatality. Insights derived from studies using non-neuronal cells have proven ineffective against neurological symptoms and the availability of pertinent cell-based models that efficiently recapitulate the HEVA71 replication cycle in neurons is sorely needed to clarify this relationship. Here, we demonstrate that HEVA71 infection of primary rat neurons and astrocytes recapitulates neuronal and astrocytic damage observed in the CNS of infected animals [15] , [16] , [17] and humans [18] , [19] , [20] . We show that viral protein VP4 triggers secretion of CXCL1 from infected astrocytes, which then acts via its receptor CXCR2 to enhance HEVA71 replication in neurons. Elevated levels of CXCL1 in cerebrospinal fluids (CSF) closely correlated with disease severity in HEVA71-infected mice, and were only detected in the CSF from severe HFMD patients with neurological complications. Using complementing strategies, we demonstrated that attenuation of neuronal CXCL1 signaling strongly suppresses viral replication. Exploiting these findings, we administered AZD5069, a selective CXCR2 antagonist, into HEVA71-infected mice and demonstrated its effectiveness in significantly lowering disease severity, extending viability and reducing viral load despite persisting elevated CXCL1 levels. Taken together, our results demonstrated that blocking CXCL1 signaling during acute HEVA71 infection can be an effective therapeutic approach to manage the effects of neuropathogenicity in severe cases of HFMD. HEVA71 efficiently and productively infects rat primary neuronal cultures There is currently no good infection model to study HEVA71 replication in CNS. Given that another Enterovirus, Coxsackievirus B3, productively infects the rat hippocampus [21] , we wondered if HEVA71 neuropathogenicity can be investigated by rat primary neuronal cultures. We exposed 7 days in vitro (DIV) cultures to two HEVA71 strains (S41 and C2) and other etiological agents of HFMD such as Coxsackievirus A6 (CA6) and Coxsackievirus A16 (CA16). S41 reportedly exhibits higher neurovirulence than C2 and other Enteroviruses [1] , [6] , [22] , [23] , [24] , [25] , [26] . At 24 h post infection (hpi), HEVA71-infected neuronal cultures revealed cytopathic effects (CPE) typically observed in other cellular models, including disintegration of neuronal processes and detachment of neuronal cell bodies (Supplementary Fig. 1a ) [26] , [27] , [28] . Consistent with the CPE, decreased cell viability was detected at 6 hpi and steadily declined, reaching below 25% by 96 hpi (Supplementary Fig. 1b ). In comparison, neuronal cultures exposed to UV-inactivated (UI) HEVA71 (controls) remained healthy throughout the monitoring period. Furthermore, neither CA6 nor CA16-infected neuronal cultures exhibited CPE or cell death (Supplementary Fig. 1c ). CPE and cell death can occur independently of productive viral infection [26] . Lack of CPE after viral infection could be attributed to lower viral infectivity [26] . To confirm if HEVA71, CA6 and CA16 replicate in neuronal cultures, we examined for the presence of viral double-stranded RNA (dsRNA), an intermediate RNA species synthesized during viral replication [4] . In parallel, neurons were stained for the neuronal microtubule-associated protein (Tau) to evaluate axonal integrity [29] . In neuronal cultures exposed to UI HEVA71, few neurons showed perinuclear dsRNA staining with axon disintegration at all time points (Fig. 1a ). In comparison, strong dsRNA signals were detected in HEVA71-infected neurons at 6 hpi when axonal disintegration also became discernible (Fig. 1a , arrowheads). In addition, approximately 80% of HEVA71-infected neurons were positive for dsRNA at 6 hpi (Fig. 1b ). These changes were also seen with HEVA71 infections at higher MOIs (Supplementary Fig. 2a ). Strikingly, neither dsRNA staining nor axon disintegration were seen in CA6 or CA16-infected neuronal cultures (Supplementary Fig. 2b ). These results indicate that, of the Enteroviruses tested here, only HEVA71 can replicate in neurons and induce CPE. Fig. 1: Productive infection     of primary neuronal cultures with HEVA71 causes neuronal cell     death. a Immunostaining of UI-, S41- or C2-infected DIV7 neuronal     cultures with antibodies against dsRNA and Tau. Scale bars     represent 20 µm. Arrowheads indicated dsRNA-positive neurons. b Quantification of     dsRNA-positive cells in infected DIV7 neuronal cultures at 6     hpi. Two hundred cells taken from random fields were manually     counted for each condition. Percentages of dsRNA-positive cells     were highest in S41- or C2-infected neurons but almost     negligible in UI-infected controls. c Immunoblotting of cell lysates from     S41-infected neuronal cultures for VP0 and VP2. β-actin was used     as a loading control. VP0 and VP2 bands appeared at 6 hpi and     continued to increase over the next 42 h. d Quantification of progeny viral particles     release into supernatants of S41- or C2-infected neuronal     cultures, where maximal viral titers were detected at 24 hpi in     DIV7 neuronal cultures. Peak viral titers were similar in both     infected neuronal cultures and RD. e Apoptotic percentages of caspase 3- or     TUNEL-positive cells were highest in S41- or C2-infected     neuronal cultures that were similar to the positive controls     (staurosporine or TAC nuclease). Two hundred cells taken from     random fields were manually counted for each condition. Scale     bars represent 20 µm. MOI of 1 was used for all experiments. Data are expressed as the average with error bars representing     ±SD from 3 independent experiments ( n = 3). Statistical analyses were performed with     two-way ANOVA corrected using Bonferroni post-test. (**** P < 0.0001). Source data are provided as a Source Data file. Full size image Productive infection of HEVA71 in infected cultures was further evidenced by the progressive rise in viral RNA and protein (VP0/VP2) levels and the release of infectious HEVA71 viral particles into the culture media (Fig. 1c, d ; Supplementary Fig. 3a ). Notably, peak viral titers were similar to those obtained from infected human rhabdomyosarcoma (RD) cells, a common cell line used for studying HEVA71 infection, albeit obtained at a slower replication rate (Fig. 1d ; Supplementary Fig. 3b ) [27] . Significant levels of apoptosis, a feature previously reported for other HEVA71 cell infection models, was also evident in HEVA71-infected neuronal cultures (Fig. 1e ; Supplementary Fig. 3c ) [30] , [31] , [32] . Interestingly, no differences in rates of replication between the S41 and C2 strains of HEVA71 were observed in neuronal cultures (Fig. 1d ; Supplementary Fig. 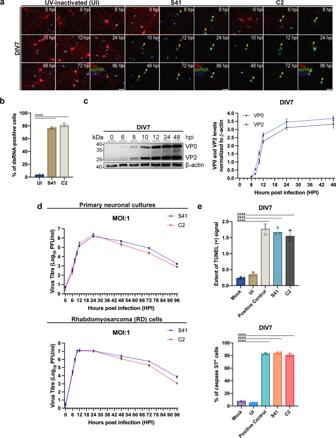Fig.     1: Productive infection     of primary neuronal cultures with HEVA71 causes neuronal cell     death. aImmunostaining of UI-, S41- or C2-infected DIV7 neuronal     cultures with antibodies against dsRNA and Tau. Scale bars     represent 20 µm. Arrowheads indicated dsRNA-positive neurons.bQuantification of     dsRNA-positive cells in infected DIV7 neuronal cultures at 6     hpi. Two hundred cells taken from random fields were manually     counted for each condition. Percentages of dsRNA-positive cells     were highest in S41- or C2-infected neurons but almost     negligible in UI-infected controls.cImmunoblotting of cell lysates from     S41-infected neuronal cultures for VP0 and VP2. β-actin was used     as a loading control. VP0 and VP2 bands appeared at 6 hpi and     continued to increase over the next 42 h.dQuantification of progeny viral particles     release into supernatants of S41- or C2-infected neuronal     cultures, where maximal viral titers were detected at 24 hpi in     DIV7 neuronal cultures. Peak viral titers were similar in both     infected neuronal cultures and RD.eApoptotic percentages of caspase 3- or     TUNEL-positive cells were highest in S41- or C2-infected     neuronal cultures that were similar to the positive controls     (staurosporine or TAC nuclease). Two hundred cells taken from     random fields were manually counted for each condition. Scale     bars represent 20 µm. MOI of 1 was used for all experiments.     Data are expressed as the average with error bars representing     ±SD from 3 independent experiments (n= 3). Statistical analyses were performed with     two-way ANOVA corrected using Bonferroni post-test.         (****P< 0.0001).     Source data are provided as a Source Data file. 3a, b ) despite the reported differences in clinical outcomes (Supplementary Table 1 ). Collectively, these results strongly support the use of primary neuronal cultures to study the mechanisms of HEVA71 neuropathogenesis. HEVA71 infection in neuronal cultures triggers massive release of CXCL1 from astrocytes HEVA71 infection elicits massive production of various cytokines [13] , [33] , [34] . However, their origins and contribution to infection outcomes in the CNS is poorly understood. 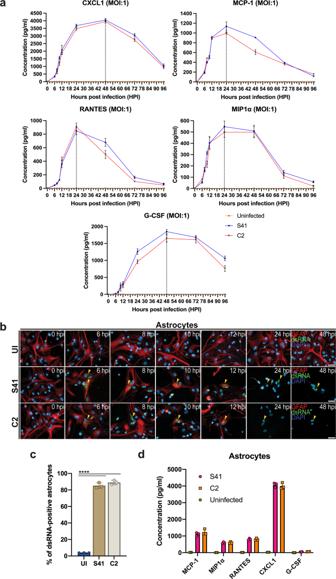Fig. 2: HEVA71 infection in     neuronal cultures induces high expression of CXCL1 with     detectable MCP-1, MIP1α and RANTES from infected     astrocytes. aLevels of the cytokines in cell culture     supernatants from S41- or C2-infected neuronal cultures     collected over a 96 h infection course. Uninfected neuronal     culture was used as control. CXCL1 showed the highest increase     during HEVA71 infection. G-CSF exhibited a delay in its     upregulation in contrast to MCP-1, MIP1α, RANTES and CXCL1.     Dotted lines represent the peak cytokine concentration that     mostly corresponded to peak viral titers detected at 24 hpi for     DIV7 neuronal cultures.bImmunostaining of S41-, C2- or UI-infected astrocytes with     antibodies against dsRNA and GFAP. Scale bars represent 20 µm.     Strong dsRNA-positive signals were detected in HEVA71-infected     astrocytes (arrowheads) but not in UI controls.cQuantification of dsRNA-positive     cells in infected astrocytes at 24 hpi. Two hundred cells taken     from random fields were manually counted for each condition.dCXCL1 was elevated in     cell culture supernatants of HEVA71-infected astrocyte cultures     but not in UI controls at 24 hpi. MOI of 1 was used for all     experiments. Data are expressed as the average with error bars     representing ±SD from 3 independent experiments (n= 3). Statistical analyses were     performed with two-way ANOVA corrected using Bonferroni     post-test. (****P< 0.0001). Source data are provided as a     Source Data file. To elucidate this, we tested culture supernatants of HEVA71-infected neuronal cultures against 23 cytokines (Supplementary Table 2 ). Of these, only 5 were highly upregulated. Four of the 5 cytokines (MCP-1, MIP1α, RANTES and CXCL1) are thought to originate from astrocytes and microglia [11] , [35] . Three of these (MCP-1, MIP1α, RANTES) peaked at time points corresponding to maximum virus production (24 hpi) (Fig. 2a ). Strikingly, highest levels of CXCL1, the most abundant cytokine detected, was sustained between 24 to 48 hpi. At higher MOIs, cytokines peaked faster, again coinciding with the timing of maximum viral titers for the respective MOIs (Supplementary Fig. 4 ). The last cytokine, neuronal G-CSF [36] , showed highest levels only at 48 hpi (Fig. 2a ). Fig. 2: HEVA71 infection in     neuronal cultures induces high expression of CXCL1 with     detectable MCP-1, MIP1α and RANTES from infected     astrocytes. a Levels of the cytokines in cell culture     supernatants from S41- or C2-infected neuronal cultures     collected over a 96 h infection course. Uninfected neuronal     culture was used as control. CXCL1 showed the highest increase     during HEVA71 infection. G-CSF exhibited a delay in its     upregulation in contrast to MCP-1, MIP1α, RANTES and CXCL1. Dotted lines represent the peak cytokine concentration that     mostly corresponded to peak viral titers detected at 24 hpi for     DIV7 neuronal cultures. b Immunostaining of S41-, C2- or UI-infected astrocytes with     antibodies against dsRNA and GFAP. Scale bars represent 20 µm. Strong dsRNA-positive signals were detected in HEVA71-infected     astrocytes (arrowheads) but not in UI controls. c Quantification of dsRNA-positive     cells in infected astrocytes at 24 hpi. Two hundred cells taken     from random fields were manually counted for each condition. d CXCL1 was elevated in     cell culture supernatants of HEVA71-infected astrocyte cultures     but not in UI controls at 24 hpi. MOI of 1 was used for all     experiments. Data are expressed as the average with error bars     representing ±SD from 3 independent experiments ( n = 3). Statistical analyses were     performed with two-way ANOVA corrected using Bonferroni     post-test. (**** P < 0.0001). Source data are provided as a     Source Data file. Full size image Neuronal cultures are known to contain some proportion of astrocytes and the finding that cytokines of astrocytic origin were released is not unexpected. Our cultures contain about 70% neurons (MAP2 + ) and 30% astrocytes (GFAP + ), similar to other reports (Supplementary Fig. 5a ) [37] . To further confirm the astrocytic origin of the cytokines, we infected highly enriched (99%; Supplementary Fig. 5b ) astrocyte cultures with HEVA71. Confirming its replication in these cultures, increasing levels of dsRNA , viral protein synthesis as well as viral particles could be detected from 6 hpi onwards (Fig. 2b, c ; Supplementary Fig. 5c–e ). Similar to other HEVA71 cell infection models [30] , [31] , [32] , infected astrocytes undergo significant apoptosis (Supplementary Fig. 5f–h ). Additionally, elevated levels of MCP-1, MIP1α, RANTES and CXCL1 were detected in culture supernatants of HEVA71-infected highly enriched astrocytes at 24 hpi similar to those seen in neuronal cultures (Fig. 2d ; Supplementary Table 2 ). Neuronal G-CSF was notably absent. Collectively, these results demonstrate that release of MCP-1, MIP1α, RANTES and CXCL1 by infected astrocytes could contribute to neuropathogenesis during HEVA71 infection. Elevation of CXCL1 in CSFs of HEVA71-infected mice and human patients correlates with clinical severity CXCL1’s level was highest amongst the elevated cytokines detected in infected neuronal and astrocyte cultures, suggesting it could strongly influence infection outcome (Fig. 2a and d ; Supplementary Table 2 ). To further determine if CXCL1 could be similarly elicited during infections in vivo, mice were infected with HEVA71 as previously described [38] . Animals intracranially infected with S41 began showing increased clinical scores and mortality from 4 dpi (Fig. 3a, b ). 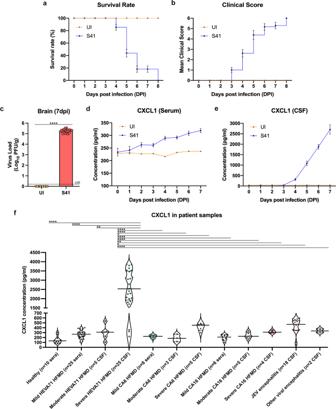Fig. 3: CXCL1     is highly detected in CSFs of HEVA71 HFMD patients and mice with     neurological deficits. aSurvival rates andbmean clinical scores of mice     infected with S41 or UI. S41-infected mice but not UI-infected     mice displayed mortality and high clinical scores from 4 dpi.cHigh viral loads were     detected in brains of S41- but not UI-infected mice (below     LOD = 0.2) at 7 dpi.d,eCXCL1 levels were     slightly elevated indserum     but highly elevated ineCSF of     S41-infected mice but not in UI-infected mice that correlated     with neuropathological deficits seen only in S41-infected mice.     Data are expressed as the average with error bars representing     ±SD from 3 independent experiments (n= 3, 10 mice were used for each group per     independent experiment).fCSF     CXCL1 chemokine concentrations in severe HEVA71 HFMD patients     significantly exceeds CXCL1 levels of other groups. Violin plots     represent all analyzed values. Bold and dashed lines indicated     median and the 25thand         75thpercentile, respectively.     Number of patients per group is indicated on thex-axis. Statistical analyses were     performed with two-way ANOVA corrected using Bonferroni     post-test. (*P< 0.05, **P< 0.01, ***P< 0.001 and ****P< 0.0001). ExactPvalues for: moderate     HEVA71 HFMD (CSF) = 0.0033, severe CA6 HFMD (CSF) = 0.0301,     severe CA16 HFMD (CSF) = 0.0038 and JEV encephalitis     (CSF) = 0.0401. Source data are provided as a Source Data     file. Noteworthy, hindlimb paralysis (indicative of HEVA71-induced CNS damage) contributed primarily to the high clinical scores documented from 4 dpi onwards (Supplementary Table 3 ) [26] . Indeed, Nissl staining revealed populations of dead neurons in both hippocampus and prefrontal cortex of S41-infected mice, coincident with the presence of viral antigens (Supplementary Fig. 6a, b ; indicated by arrowheads). Furthermore, high viral titers could be measured (Fig. 3c ). Meanwhile, UI-infected mice exhibited none of these adverse features. Thus, HEVA71 replication in the brains of these mice contributes to CNS damage and eventual death. Fig. 3: CXCL1     is highly detected in CSFs of HEVA71 HFMD patients and mice with     neurological deficits. a Survival rates and b mean clinical scores of mice     infected with S41 or UI. S41-infected mice but not UI-infected     mice displayed mortality and high clinical scores from 4 dpi. c High viral loads were     detected in brains of S41- but not UI-infected mice (below     LOD = 0.2) at 7 dpi. d , e CXCL1 levels were     slightly elevated in d serum     but highly elevated in e CSF of     S41-infected mice but not in UI-infected mice that correlated     with neuropathological deficits seen only in S41-infected mice. Data are expressed as the average with error bars representing     ±SD from 3 independent experiments ( n = 3, 10 mice were used for each group per     independent experiment). f CSF     CXCL1 chemokine concentrations in severe HEVA71 HFMD patients     significantly exceeds CXCL1 levels of other groups. Violin plots     represent all analyzed values. Bold and dashed lines indicated     median and the 25 th and         75 th percentile, respectively. Number of patients per group is indicated on the x -axis. Statistical analyses were     performed with two-way ANOVA corrected using Bonferroni     post-test. (* P < 0.05, ** P < 0.01, *** P < 0.001 and **** P < 0.0001). Exact P values for: moderate     HEVA71 HFMD (CSF) = 0.0033, severe CA6 HFMD (CSF) = 0.0301,     severe CA16 HFMD (CSF) = 0.0038 and JEV encephalitis     (CSF) = 0.0401. Source data are provided as a Source Data     file. Full size image To examine if CXCL1 is released upon infection of these animals, we assayed sera and CSF collected from S41- or UI-infected mice from 0 to 7 dpi. In S41-infected mice, serum CXCL1 levels rose slightly but CSF levels of the chemokine rapidly increased from 4 dpi onwards (Fig. 3d, e ). This coincided temporally with the onset and progressive worsening of mortality and clinical scores in these animals. Of note, no changes were observed in CXCL1 levels in sera or CSF of UI controls throughout the 7 day monitoring period (Fig. 3d, e ). To further clarify the source of CXCL1, we stained neuronal cultures against CXCL1 in combination with Tau (neurons) or GFAP (astrocytes). Only infected dsRNA-positive astrocytes expressed CXCL1 (Supplementary Fig. 7 , indicated by arrows). Confirming this, only astrocytes in brains of S41-infected mice expressed CXCL1 while the chemokine was noticeably absent in neurons (NeuN + ) and microglia (IBA1 + ) (Supplementary Fig. 8a, b ; indicated by arrowheads). Meanwhile, CXCL1 was not detected in all 3 cell types in UI controls. CXCL1 is a known chemoattraction for neutrophils [39] , [40] . We further examined if the observed neuropathology could be caused by infiltrating neutrophils as reported in other viral infections [41] , [42] , [43] . Neonatal mice were intracranially infected with HEVA71 as before and then treated with isotype IgG (IgG) or anti-Ly6G antibodies (Ly6G-Ab) [44] , [45] at 1 mg/kg once daily till 5 dpi. Progressive mortality and increase in clinical scores were similar between IgG- and Ly6G-Ab-treated S41-infected mice, as were viral titers at 7 dpi (Supplementary Fig. 9a–c ). Likewise, similar increase in CSF CXCL1 levels occurred from 4 dpi onwards in both groups of S41-infected mice while sera CXCL1 levels remain unchanged (Supplementary Fig. 9d, e ). As expected, UI controls remained healthy and no changes in CXCL1 levels were seen throughout the monitoring period (Supplementary Fig. 9a–e ). Fluorescence-activated cell sorting analyses (FACS) of dissociated cells from infected brain areas doubly labeled for CD45 and Ly6G, markers for neutrophils, showed very low neutrophil infiltration into these areas even in the absence of treatment with anti-Ly6G antibodies (Supplementary Fig. 9f ). In comparison, FACS of infected hindlimb muscles from the same animals contained elevated populations of these cells (Supplementary Fig. 9f ). Taken together, these results demonstrate that neutrophils do not contribute to CNS damage during HEVA71 infection and reinforces the release of CXCL1 from astrocytes as an important cause of CNS damage and eventual mortality. CXCL1 release in HFMD patients has not been studied. We measured CXCL1 levels in sera and CSFs obtained from healthy individuals, patients suffering from non-HFMD-related viral infections (JEV) with CNS neurological complications [46] , as well as from HFMD patients (HEVA71, CA6 or CA16) exhibiting varying degrees of clinical severity [47] , [48] . All were under 65 months of age at the point of infection (Supplementary Fig. 10 ). Only CSFs from severe HEVA71 HFMD patients contain significantly elevated CXCL1 levels (Fig. 3f ), which were similar to those detected in our infected neuronal cultures and mice. Supporting our earlier findings that CA6 and CA16 did not infect neurons, only low levels of CSF CXCL1 were present in patients severely infected by these viruses. Thus, elevated levels of CXCL1 is strongly linked to the neuropathogenesis observed in severe HEVA71 infections in humans. CXCL1 enhances HEVA71 replication in neuronal cultures CXCL1 binds to the neuronal CXCR2 receptor to activate downstream extracellular signal-regulated kinase 1/2 (ERK1/2) in neurons during neurodevelopment and neural repair [49] , [50] . Intriguingly, phosphorylated ERK1/2 (pERK1/2) has been paradoxically reported to both enhance HEVA71 replication [51] and initiate antiviral and anti-apoptotic responses; the latter in cooperation with Janus kinase 2 (JAK2) to phosphorylate STAT3 at its serine 727 (pS727) and tyrosine 705 (pT705) residues [52] , [53] . The strong correlation of CXCL1 levels with disease severity is striking and indicated that the cytokine could promote viral infection. To discriminate between the 2 contrasting roles, we exposed neurons to CXCL1 prior to infection. Pre-treatment of neurons with 25 units (U) or more of CXCL1 both accelerated and increased viral titers at 12 hpi in comparison to untreated controls (Fig. 4a ). Expectedly, these were accompanied by an earlier drop in viral titer and a faster decline in neuronal viability (Supplementary Fig. 11a ). Production of viral proteins was similarly enhanced. Significantly higher levels of VP0 and VP2 were observed at 12 hpi instead of 24 hpi as seen in untreated controls (Fig. 4b , lanes 4, 7 and 10 versus lane 2; Fig. 4c ). Fig. 4: CXCL1 signaling activates     downstream ERK1/2 via CXCR2 to enhance viral replication in     neuronal cultures. a HEVA71 viral titers increase in     CXCL1-pretreated DIV7 neuronal cultures. Exact P values for: 25 U/ml at 24 hpi =     0.0033 and 48 hpi = 0.0009. b Immunoblotting of cell lysates from CXCL1-pretreated or     untreated S41-infected DIV7 neuronal cultures against VP0, VP2,     ERK1/2, pERK1/2, JAK2, pS727 (STAT3), pT705 (STAT3) and STAT3. CXCL1 pre-treatment accelerates the appearance HEVA71 viral     proteins. Elevated pERK1/2 and ERK1/2 levels also emerged     earlier. Immunoblot representative of 3 biological repeats is     shown. Bar charts below show the quantifications for each     protein. c High levels of VP0     and VP2 were detectable at 12 hpi only with exposure to CXCL1. Exact P values for VP0: 25     U/ml at 24 hpi = 0.0195, 50 U/ml at 24 hpi = 0.0001 and 100 U/ml     at 24 hpi = 0.002. Exact P values for VP2: 25 U/ml at 24 hpi = 0.001 and 100 U/ml at 24 hpi     = 0.0215. d pERK1/2 to ERK1/2     ratios were higher in pretreated cultures versus controls in a     CXCL1 dose-dependent manner at all timepoints. Exact P value for pERK1 to ERK1 ratio: 25     U/ml at 48 hpi = 0.0094. β-actin was used as a loading control     for immunoblotting experiments. MOI of 1 was used for all     experiments. Data are expressed as the average with error bars     representing ±SD from 3 independent experiments ( n = 3). Statistical analyses were     performed with two-way ANOVA corrected using Bonferroni     post-test. (* P < 0.05, ** P < 0.01, *** P < 0.001 and **** P < 0.0001). Source data     are provided as a Source Data file. Full size image An earlier and higher phosphorylation of ERK1/2 and STAT3(pS727) coincided with the accelerated viral replication in CXCL1 pre-treated neurons (Fig. 4b , lanes 4, 7 and 10 versus lane 1; Fig. 4d ; Supplementary Fig. 11b, c ). Furthermore, absence of JAK2 and STAT3(pT705) in both untreated and CXCL1-pretreated neuronal cultures at time points after peak viral protein production argues against the involvement of pERK1/2 in initiating anti-viral responses via JAK2 (Fig. 4b , lanes 2-12; Supplementary Fig. 11d ). Neuronal apoptosis coinciding with the timing of higher pERK1/2 levels also supports the role of the latter in enhancing viral replication (Fig. 1e ). To further confirm that CXCL1 acts via the CXCR2-ERK1/2 pathway to enhance viral replication, we demonstrated that ERK1/2 activation can be blocked by its selective inhibitor FR180204 in CXCL1-treated uninfected neurons (Supplementary Fig. 12a, b ) [54] . Single application of FR180204 to these infected neurons decreased viral titers (Fig. 5a ), reduced neuronal death (Supplementary Fig. 12c ) and lowered viral protein expression together with ERK1/2 activation as compared to vehicle-treated controls at 12 and 24 hpi (Fig. 5b , lanes 1-2 versus lanes 4-5; Fig. 5c, d ; Supplementary Fig. 12d ). FR180204 has a reported half-life of 36 h [55] and viral protein synthesis could be observed to progressively resume by 24 hpi in FR180204-treated neurons (Fig. 5b , lanes 5-6; Fig. 5c ). Notably, levels of JAK2 and STAT3(pT705) persisted when phosphorylation of ERK1/2, STAT3(pS727) remained low but progressively declined upon activation of ERK1/2 (Fig. 5b , lanes 4-6; Supplementary Fig. 12e, f ). Fig. 5: Blocking CXCL1 signaling     by pERK1/2 inhibition reduces viral replication in neuronal     cultures. a Inhibiting ERK1/2 decreased viral titers at 12     and 24 hpi in DIV7 neuronal cultures. b Immunoblotting of S41-infected DIV7 neuronal     cultures treated simultaneously with FR180204 (5 µM) and CXCL1     (100 U/ml) at 12, 24 and 48 hpi. ERK1/2 inhibition delays the     expression of HEVA71 viral proteins. Immunoblot representative     of 3 biological repeats is shown. Bar charts below show the     quantifications for each protein. c VP0 and VP2 levels decreased at 12 and 24 hpi     with ERK1/2 inhibition. d pERK1/2 to ERK1/2 ratios were reduced at all timepoints in     FR180204-treated cultures. Exact P value for pERK1 to ERK1 ratio with FR180204 at     48 hpi = 0.0001. β-actin was used as a loading control for     immunoblotting experiments. MOI of 1 was used for all     experiments. Data are expressed as the average with error bars     representing ±SD from 3 independent experiments (n = 3). Statistical analyses were performed with two-way ANOVA corrected     using Bonferroni post-test. (*** P < 0.001 and **** P < 0.0001). Source data     are provided as a Source Data file. Full size image We then validated these results using another approach by deleting the CXCR2 gene using lentiviral-mediated CRISPR/Cas9 to test whether removal of the receptor could also affect CXCL1-mediated enhancement of viral replication. CXCR2 expression in neuronal cultures was almost completely abolished via gene editing with CXCR2 sgRNAs (Supplementary Fig. 13a ). In agreement with the observations using pharmacological inhibition of ERK1/2 activation, CXCR2 deficiency significantly reduced viral titer (Fig. 6a ), neuronal death (Supplementary Fig. 13b ) and viral protein expression in CXCL1-pretreated infected neuronal cultures ( CXCR2 sgRNA) as compared to similarly pretreated infected control neuronal cultures LOC116160065 ( LUC sgRNA) (Fig. 6b , lanes 1-3 versus lanes 4-6; Fig. 6c ). Lower levels of ERK1/2 activation were also detected, supporting that CXCR2 is necessary for ERK1/2 phosphorylation (Fig. 6b , lanes 1-3 versus lanes 4-6; Fig. 6d ; Supplementary Fig. 13c ). Moreover, JAK2 and STAT3(pT705) remained detectable in infected CXCR2-deficient neuronal cultures (Fig. 6b , lanes 4-5; Supplementary Fig. 13d, e ). Fig. 6: Blocking CXCL1 signaling     by CXCR2 deletion decreases viral replication in neuronal     cultures. a CXCR2 deletion in infected neuronal cultures reduced viral titers at     all time points tested. b Lysates from neuronal cultures infected with control ( LUC sgRNA)- or CXCR2 sgRNA-expressing lentiviruses were     similarly immunoblotted as in a . CXCR2 deletion     delays viral protein expression in neuronal cultures despite     CXCL1 pretreatment. Immunoblot representative of 3 biological     repeats is shown. Bar charts below show the quantifications for     each protein. c VP0 and VP2     levels decreased at all timepoints in CXCR2 -deleted samples. d pERK1/2 to ERK1/2 ratios were decreased in CXCR2 -deleted samples. β-actin was used as a loading control for immunoblotting     experiments. MOI of 1 was used for all experiments. Data are     expressed as the average with error bars representing ±SD from 3     independent experiments ( n = 3). Statistical analyses were performed with     two-way ANOVA corrected using Bonferroni post-test. (**** P < 0.0001). Source data are provided as a Source Data file. Full size image Further supporting its involvement in enhancing viral replication only in neurons of neuronal cultures, CXCL1 pre-treatment did not accelerate viral replication, neuronal death, ERK1/2 activation and JAK2 degradation in infected astrocytes (Supplementary Fig. 14a–e ), which do not express CXCR2 (Supplementary Fig. 14f ). Surprisingly, viral synthesis and ERK1/2 activation increased in neuronal cultures at 48 hpi and was accompanied by strong reduction of JAK2 and STAT3(pT705) (Fig. 6b , lane 6; Fig. 6c, d ; Supplementary Fig. 13c–f ). This suggested that residual CXCL1 signaling through incompleted knockout of CXCR2 could eventually still allow viral replication to continue. Collectively, the results confirmed that astrocytic CXCL1 acts directly on neuronal CXCR2 to enhance viral replication in neurons. HEVA71 VP4 elicits CXCL1 release and is required for viral replication in neurons Next, we wondered which viral protein(s) could trigger CXCL1 release. EGFP-tagged viral protein (VP1 to VP4, 2A to 2C, 3A to 3D) or EGFP alone (control) were individually expressed lentivirally in neuronal cultures and astrocytes (Supplementary Fig. 15a, b ). CXCL1 assays at 6 dpi indicated only VP4 was able to increase CXCL1 levels in both cultures (Fig. 7a ; Supplementary Fig. 15c ). Incidentally, neurons expressing VP4 exhibited cell death whereas viral 3C protease (3C pro ) was responsible for astrocytic cell death (Supplementary Fig. 15a, b ). None of the other viral proteins tested showed similar effects. Fig. 7: HEVA71 VP4 induces     CXCL1 secretion for HEVA71 replication and subsequent viral     neuropathogenesis in neuronal         cultures. a CXCL1 levels were elevated in culture     supernatants when VP4 and VP4-mut were expressed. Higher levels     of the chemokine were detected in samples expressing wildtype     VP4. b Immunofluorescence     images of control (EGFP)- or VP4 (wildtype and mutant)-     expressing neuronal cultures. Neurite disintegration was only     observed in wildtype VP4-expressing neuronal cultures. Scale     bars represent 20 µm. c Immunoblots of cell lysates from control (EGFP)-, VP4- or     VP4-mut-expressing neurons against VP4, EGFP, ERK1/2, pERK1/2,     pS727 (STAT3), JAK2, pT705 (STAT3), STAT3, caspase 3 and cleaved     caspase 3. Immunoblot representative of 3 biological repeats is     shown. Bar charts below show quantifications for each protein. d pERK1/2 to ERK1/2 ratios     were higher in VP4-expressing neuronal cultures as compared to     VP4-mut or EGFP controls at all time points. e Cleaved caspase 3 was detected only     in VP4-expressing neuronal cultures. Exact P value for caspase 3: VP4-mut at 6     dpi = 0.6026. β-actin was used as a loading control for     immunoblotting experiments. Data are expressed as the average     with error bars representing ±SD from 3 independent experiments         ( n = 3). Statistical     analyses were performed with two-way ANOVA corrected using     Bonferroni post-test. (ns > 0.9999 unless specified, and         **** P < 0.0001). Source data are provided as a Source Data file. Full size image Myristoylation, a covalent attachment of a 14-carbon saturated fatty acid, the myristate group, to the N-terminal glycine (G) of VP4 , is essential for proper VP4 function in HEVA71 replication [56] , [57] , [58] . We mutated glycine at position 2 of its N-terminal myristoylation motif (M G XXXS) to alanine (M A XXXS) in order to render it myristoylation-deficient (VP4-mut) (Supplementary Fig. 15d ). This was confirmed by the absence of myristylation using a myristoylation-specific antibody in VP4-mut immunoprecipitated from neuronal lysates (Supplementary Fig. 15e, f ). Expressing EGFP-tagged VP4-mut alone in neuronal cultures and astrocytes strongly reduced CXCL1 production as compared to wildtype VP4 (Fig. 5a ; Supplementary Fig. 15c ). Moreover, neurons expressing VP4-mut appeared viable (as did astrocytes) (Fig. 7b ; Supplementary Fig. 15g ). Given the diminished ability of VP4-mut to stimulate CXCL1 release and cause neuronal cell death, we wondered if VP4-mut could inhibit infectivity of HEVA71 viruses carrying this mutation. We observed that ERK1/2 was not phosphorylated in astrocytes expressing either form of VP4 (Supplementary Fig. 15h ). Instead, pERK1/2 could clearly be detected in neuronal cultures (Fig. 7c, d ). Moreover, similar to their differences in eliciting CXCL1 release, VP4-mut was less potent at causing phosphorylation of ERK1/2 (and also downstream STAT3-pS727) as compared with wildtype VP4 (Fig. 7c, d ; Supplementary Fig. 15i, j ). Only VP4 was able to induce elevation in ERK1/2 levels, which was not seen with VP4-mut or EGFP expression (Supplementary Fig. 15i ). Additionally, VP4-mut expression did not cleave caspase 3 whereas wildtype VP4 triggered robust caspase 3 cleavage (Fig. 7c and e ). Notably, expression levels of both VP4 variants were similar to those observed in infections using whole virions (Supplementary Fig. 15k, l ). This indicated that these findings were not due to over-expression artefacts. Moreover, only 3C pro (not either of the VP4 variants) triggered caspase 3 cleavage when singly expressed in astrocytes (Supplementary Fig. 15m ). These results reiterate the specificity of VP4-induced CXCL1 signaling in neurons. To determine if VP4 mutations indeed attenuate HEVA71 infection in neurons, we generated VP4-mutant HEVA71 viruses using an infectious clone [59] , [60] . In human RD cells, both wildtype and VP4-mut viruses displayed similar viral fitness (viral replication, translation and peak viral titer) (Supplementary Fig. 16 ). VP4-mut viruses were significantly attenuated in infecting neuronal cultures in contrast to their wildtype counterparts. VP4-mut viruses displayed a long lag in viral protein synthesis and took a significantly longer time to reach peak viral titers similar to wildtype viruses (>144 versus 24 hpi) (Supplementary Fig. 17 ). Likewise, CXCL1 levels from VP4-mutant virus infected cultures took 6 times longer (144 versus 24 hpi) to reach similar levels elicited by wildtype viruses—something that was not observed in infected RD cells (Supplementary Fig. 18 ). The lower extent of CXCL1 production commensurated with reduced viral protein synthesis and pERK1/2 levels, accompanied by detection of JAK2 and STAT3(pT705) in VP4-mutant HEVA71-infected cultures in contrast to their wildtype counterparts (Fig. 8a–c ; Supplementary Fig. 19a, b ). Of note, ERK1/2 levels were also lower in VP4-mutant HEVA71-infected cultures than in wildtype cultures, agreeing with our previous results using lentiviral VP4 expression (Supplementary Fig. 19c ). Fig. 8: VP4-mutant HEVA71     reduces CXCL1 signaling and subsequent HEVA71 replication in     neuronal cultures. a Immunoblots of cell lysates from wildtype     HEVA71 and VP4-mutant HEVA71-infected DIV7 neuronal cultures at     12, 24 and 48 hpi. Similar primary antibodies excluding caspase     3 were used. VP4 mutation delays the expression of HEVA71 viral     proteins. Immunoblot representative of 3 biological repeats is     shown. Bar charts below show quantifications for each protein. b VP0 and VP2 levels     decreased at all time points in neurons infected with VP4-mutant     HEVA71. Exact P values for:     VP0 at 48 hpi = 0.018 and VP2 at 48 hpi = 0.0161. c pERK1/2 levels were decreased in     VP4-mutant HEVA71-infected neurons. Data are expressed as the     average with error bars representing ±SD from 3 independent     experiments ( n = 3). Statistical analyses were performed with two-way ANOVA corrected     using Bonferroni post-test. (* P < 0.05 and **** P < 0.0001). Source data are provided as     a Source Data file. Full size image Reverting to our mice model, we intracranially infected animals with wildtype, VP4-mut or UI viruses and monitored them afterwards for 15 days. Supporting our in vitro observations, mortality and the onset of clinical manifestations were significantly delayed in VP4-mut virus-infected mice (7 dpi) whereas they appeared earlier (3 and 4 dpi, respectively) in wildtype virus-infected mice (Fig. 9a, b ). These changes were accompanied by significantly lower viral loads in the brains of VP4-mut versus wildtype infected mice at 7 dpi (Fig. 9c ). Moreover, CSF levels of CXCL1 in VP4-mut infected mice remained undetectable until after 6 dpi (versus 4 in wildtype) and only reached equivalent highest levels around 13 dpi (versus around 7 dpi in wildtype) (Fig. 9d ). Only slight differences in sera CXCL1 levels were observed in mice infected with either virus (Fig. 9e ). Interestingly, the delayed onset of CXCL1 secretion, severe clinical manifestations and mortality in VP4-mut versus wildtype infected mice was not due to the reversion of VP4-mut to its wildtype counterpart virus (Supplementary Fig. 20 ). For both viruses, detection of CXCL1 preceded the onset of clinical symptoms and fatality. Notably, no change was observed in sera or CSF CXCL1 levels of UI controls throughout 15 dpi, which is in agreement with the negligible viral titers, lack of fatality and clinical symptoms (Fig. 9a–e ). Fig. 9: Mutating HEVA71 VP4     reduces CXCL1 signaling and associated HEVA71 replication and     neuropathogenesis in mice. a – e Infection of mice with wildtype or VP4-mutant     HEVA71 virons. a Survival rates     and b mean clinical scores of     mice infected with wildtype, VP4-mutant or UI virus. Wildtype     and VP4-mutant HEVA71-infected mice displayed mortality and high     clinical scores from 4 and 7 dpi, respectively. UI-infected mice     were healthy till 15 dpi. c VP4-mutant HEVA71-infected mice had lower viral loads detected     in their brains at 7 dpi. UI-infected mice were used as     controls. Negligible viral loads were detected below limit of     detection (LOD = 0.2). d , e CXCL1 levels were highly     elevated in d CSF but only     slightly elevated in e serum of     both wildtype and VP4-mutant HEVA71-infected mice but not in     UI-infected mice. Wildtype HEVA71-infected mice showed     increasing CXCL1 from 4 dpi but those for VP4-mutant-infected     mice emerged at 7 dpi. f Brain     lysates of wildtype, VP4-mutant or UI-infected mice were     analyzed by immunoblotting at 7 dpi. Infection with VP4-mutant     HEVA71 delays the expression of HEVA71 viral proteins. Immunoblot representative of 3 biological repeats is shown. Bar     charts below show quantifications for each protein. g VP0 and VP2 levels decreased at 7     dpi with VP4-mutant HEVA71. Exact P values for: VP0 = 0.0009 and VP2 = 0.0002. h pERK1/2 were reduced in     VP4-mutant HEVA71-infected mice. Exact P values for: pERK1 = 0.0009 and pERK2 = 0.0012. i Cleaved caspase 3 was     detected in wildtype HEVA71-infected mice but not VP4-mutant     HEVA71-infected mice at 7 dpi. Exact P values for: caspase 3 = 0.0254 and cleaved     caspase 3 = 0.0008. β-actin was used as a loading control for     immunoblotting experiments. Data are expressed as the average     with error bars representing ±SD from 3 independent experiments         ( n = 3). Statistical     analyses were performed with two-way ANOVA corrected using     Bonferroni post-test. (** P < 0.01, *** P < 0.001 and **** P < 0.0001). Source data     are provided as a Source Data file. Full size image The improved infection outcome observed in VP4-mut infected mice corroborated with lower synthesis of viral proteins, less phosphorylation of ERK1/2 along with lower ERK1/2 levels as well as negligible cleavage of caspase 3 at 7 dpi as compared to wildtype infected mice (Fig. 9f–i ; Supplementary Fig. 21a ). Likewise, JAK2 and STAT3(pT705) levels persisted in VP4 mutant HEVA71-infected mice (Fig. 9f ; Supplementary Fig. 21b, c ). As expected, viral proteins, pERK1/2 and cleaved caspase 3 were undetectable in UI-infected animals (Fig. 9f–i ). Taken together, the results presented demonstrate that perturbing VP4 function significantly attenuates HEVA71 infection in neurons, thereby significantly reducing neuropathogenesis. Suppressing CXCL1 signaling with AZD5069 prolongs survival and reduces clinical severity in HEVA71-infected mice Given the critical involvement of CXCL1 in establishing neuronal infections, we wanted to evaluate whether pharmacological pertubation of its signaling would interfere with and, hence, alleviate HEVA71-induced neuropathogenesis. AZD5069, a drug currently used for cancer and respiratory illness in humans, is a potent, selective and reversible CXCR2 antagonist [61] , [62] . Indeed, application of AZD5069 to CXCL1-exposed neuronal cultures effectively reduced ERK1/2 activation with no observable toxicity (Supplementary Fig. 22a, b ). Single application of AZD5069 to infected neuronal cultures reduced pERK1/2 levels and delayed viral protein synthesis by at least 12 h in contrast to vehicle-treated controls (Supplementary Fig. 22c , lanes 1-2 versus lanes 4-5; Supplementary Fig. 22d, e ). AZD5069 has a reported half-life of 16 h [61] . In agreement with this, viral protein synthesis and increased pERK1/2 levels resumed from 24 hpi, accompanied by the gradual disappearance of JAK2 and STAT3(pT705) (Supplementary Fig. 22c , lanes 5-6; Supplementary Fig. 22d–g ). Together, these results showed that a single dose of AZD5069 is already sufficient to interrupt and delay the replication of HEVA71 in neurons. To assess if AZD5069 can improve infection outcome in vivo, we intracranially administered AZD5069 (10 mg/kg) or vehicle control (PBS) once every 2 days up till 5 dpi in our HEVA71-infected mouse model. Strikingly, mortality and the onset of clinical symptoms were siginficantly delayed in AZD5069-treated infected mice as compared to vehicle control (7 and 8 dpi versus 3 and 4 dpi, respectively) (Fig. 10a, b ). Concomitant with the milder infection in AZD5069-treated mice, much lower viral titers in the brain were detected between 4 to 7 dpi as opposed to those treated with vehicle control (Fig. 10c ). Fig. 10: Suppressing CXCL1     signaling by AZD5069 treatment improved survival and clinical     scores that correlated with reduced HEVA71 viral load in     infected mice. a Survival rates and b mean clinical scores of mice infected with S41     or UI with or without AZD5069 treatment, respectively. Arrowheads indicate time points of AZD5069 administration. S41-infected mice displayed mortality and high clinical scores     from 4 dpi. AZD5069 administration to S41-infected mice delayed     mortality and high clinical scores until 8 dpi. UI-infected mice     were healthy till 15 dpi. c AZD5069 treatment lowered viral loads in brains of S41-infected     mice from 4 to 7 dpi. d , e CXCL1 levels were     slightly elevated in d serum     but highly elevated in e CSF of     S41-infected mice with or without AZD5069 but not in UI-infected     mice. f Brain lysates of S41-     or UI-infected mice with or without AZD5069 treatment were     subjected to immunoblotting analyses at 7 dpi. AZD5069 treatment     delays the expression of HEVA71 viral proteins. Immunoblot     representative of 3 biological repeats is shown. Bar charts     below show quantifications for each protein. g VP0 and VP2 levels decreased at 7     dpi with AZD5069 treatment. Exact P values for: VP0 = 0.0006 and VP2 = 0.0009. h pERK1/2 and ERK1/2 levels     were reduced in AZD5069-treated mice. Exact P values for: ERK1 = 0.0002,     ERK2 = 0.0013, pERK1 = 0.0001 and pERK2 = 0.0007. i JAK2 levels persisted in     CXCR2-suppressed mice with S41 infection. Exact P values for: JAK2 = 0.001. j AZD5069 treatment     increased phosphorylation of STAT3 at pT705 but decreased pS727     levels at 7 dpi. Exact P values for: pT705 = 0.0007. k Cleaved caspase 3 was detected only in S41-infected mice without     AZD5069 treatment at 7 dpi. Exact P values for: caspase 3 = 0.0013 and cleaved     caspase 3 = 0.0015. β-actin was used as a loading control for     immunoblotting experiments. Data are expressed as the average     with error bars representing ±SD from 3 independent experiments         ( n = 3). Statistical     analyses were performed with two-way ANOVA corrected using     Bonferroni post-test. (** P < 0.01, *** P < 0.001 and **** P < 0.0001). Source data     are provided as a Source Data file. Full size image Levels of CXCL1 in the sera and CSF did not differ between the treated and untreated groups (Fig. 10d, e ), indicating that AZD5069 had no effect on CXCL1 release. Yet, immunoblotting of brain lysates revealed that AZD5069-treated infected mice showed reduced levels of viral protein synthesis and phosphorylated pERK1/2 in comparison to vehicle-treated controls at 7 dpi (Fig. 10f , lane 2 versus lane 1; Fig. 10g, h ). Likewise, caspase 3 cleavage was absent in AZD5069-treated infected mice, and JAK2 and STAT3(pT705) remained detectable (Fig. 10f , lane 2 versus lane 1; Fig. 10i–k ). Of note, the detection of low percentages of CD45- and Ly6G-positive neutrophils in brains of both AZD5069- and PBS-treated infected mice at 7 dpi affirmed that reduced CNS damage upon AZD5069 treatment was not due to blockage of CXCL1-mediated neutrophil recruitment into CNS (Supplementary Fig. 23 ). AZD5069 was not effective at curbing mortality, high clinical scores, viral loads and CXCL1-mediated signaling axis when given intravenously in S41-infected mice (Supplementary Fig. 24 ), suggesting that AZD5069 was unable to cross the blood-brain barrier to enter the CNS and prevent CXCL1-mediated HEVA71 neuropathogenesis. Collectively, these results demonstrate that targeting CXCL1 signaling during severe HEVA71 infections is a viable strategy to limit neutrophil-independent CNS damage and improve infection outcome. Dysregulated cytokine production is strongly linked to severe HEVA71 infections with neurological complications [9] . However, the identity of CNS relevant cytokines and how they contribute to severe infections remain obscure [63] , [64] , [65] . We showed that productive HEVA71 infection of neurons and astrocytes elicits release of a subset of cytokine and chemokines. Of these, elevated levels of CXCL1 are detected only in patients suffering from severe HFMD involving neurological complications. CXCL1, released from infected astrocytes by VP4, activates its neuronal receptor CXCR2 to phosphorylate downstream ERK1/2 that, in turn, promotes HEVA71 replication in neurons (Supplementary Fig. 25 ). Perturbation of CXCL1 signaling using 2 distinct pharmacological strategies and, independently, via a genetic approach in vitro and in vivo effectively reduced viral replication while also preventing neuronal cell death and improving infection outcome. AZD5069 treatment of HEVA71-infected mice delayed mortality and the onset of clinical symptoms (Supplementary Fig. 26 ). Collectively, these results uncover the involvement of CXCL1 in causing neurological complications and highlight the feasibility of pharmacologically interfering its signaling in the treatment of severe HFMD infections. Whilst low CXCL1 levels in sera were previously detected in HFMD patients, its levels in CSF and relation to disease severity has not been hitherto appreciated [66] . Our study demonstrates the chemokine’s involvement as a neuronal specific pro-viral factor to promote HEVA71’s infection in neurons. Although CXCL1 has been reported to facilitate CNS infiltration of neutrophils during mouse hepatitis virus (JHMV) [41] , West Nile virus (WNV) [42] and herpes simplex virus 1 (HSV1) infections [43] , our results revealed the lack of contribution by CXCL1-recruited infiltrating neutrophils in causing HEVA71-induced CNS damage. Indeed, this is consistent with previous reports showcasing sparse neutrophil presence in CNS during HEVA71 infection [67] , [68] , [69] , even though some studies have reported otherwise [70] , [71] . Despite this controversy, our additional observations that neuronal cell death occurs in our cultures in the absence of neutrophils and that CXCL1 directly enhances viral replication in neurons, strongly indicate viral replication but not neutrophils as the primary cause of damage. The structural protein VP4 is known to participate in viral entry [72] , [73] . However, the possibility of its involvement in directly targeting host functions during enteroviral infections has not been reported. We observe that VP4 expression in astrocytes is sufficient to trigger the release of large amounts of CXCL1 from these cells. Myristylation-deficient VP4, while still capable of eliciting lower amounts of CXCL1 release, attenuated HEVA71’s ability to infect neurons. These findings are significant as they established a role for VP4 as a proviral factor important for establishing HEVA71 infections in the CNS. Understanding how VP4 regulates astrocytic CXCL1 expression and how it promotes HEVA71 replication in neurons but not other cells are topics requiring further investigation. Expression of CXCR2 in neurons but not astrocytes and release of CXCL1 in the latter but not former indicates an unidirectional axis of signaling for CXCL1 from astrocytes to neurons during the course of virus infection. Indeed, perturbing this signaling disrupts HEVA71 replication in neurons but not astrocytes. CXCL1 and CXCR2 have been implicated in other forms of CNS injury and blockade of CXCR2 signaling has been shown to be neuroprotective [74] . In agreement with previous studies, activation of CXCR2 in neurons increased ERK1/2 phosphorylation [75] . Activated ERK1/2 is required for enhancing viral replication [51] , [76] . Supporting this, VP4-mut HEVA71 viruses that were less competent at eliciting CXCL1 release and ERK1/2 phosphorylation exhibited lower rates of replication. This is in agreement with the notion that ERK1/2 activation must exceed a certain threshold before HEVA71 can efficiently infect neurons [57] , [58] . Elevated ERK1/2 activation can also promote apoptosis. Indeed, previous studies observed positive correlation between pERK1/2 levels with neuronal death in neurodegenerative diseases [77] . The VP4-CXCL1-CXCR2-ERK1/2 axis appears to be the predominant if not sole mechanism for triggering neuronal but not astrocyte apoptosis. Supporting this, VP4-mut, which was significantly less able to activate ERK1/2, could not induce neuronal apoptosis. In comparison, viral 3C pro expression induces astrocyte but not neuronal apoptosis, possibly by activating caspase 8 as shown in other studies [30] , [78] . Thus, coordination between different viral and host proteins may be required to regulate apoptosis in different cell types during viral infection. Apart from ERK1/2 activation, our study documented significant ERK1/2 upregulation during HEVA71 replication in neuronal cultures, particularly during VP4 presence. Reinforcing this notion, VP4-mut was found to maintain basal ERK1/2 levels in neuronal cultures. As previously reported, many viruses along with HEVA71, such as human immunodeficiency virus (HIV), hepatitis C virus (HCV) and Kaposi’s sarcoma-associated herpesvirus (KSHV) can target ERK1/2 pathways as a means to manipulate cellular function and to regulate viral infection and replication, albeit it should be noted that ERK1/2 activation rather than its upregulation was documented in those studies [79] , [80] , [81] , [82] . Given that ERK1/2 elevation was not present in infected astrocytes, we can only suspect that myristoylated VP4 could cause ERK1/2 accumulation specifically in neurons, which would require further investigation. The lack of a HEVA71 vaccine has prompted intense studies to identify effective antivirals against severe HEVA71 infections [4] . We showed that AZD5069, a reversible and selective CXCR2 antagonist, efficiently inhibited viral replication and significantly improved clinical severity and survival rates in HEVA71-infected mice. AZD5069 is safe and well-tolerated in humans and is currently in used for the treatment of several diseases [83] , [84] , [85] . However, our results demonstrating the poor permeability of intravenously administered AZD5069 along with its documented low bioavailability across blood-brain barrier following oral administration [86] limits its direct application against HEVA71 pathogenesis. Testing AZD5069 derivatives that can effectively cross the blood-brain barrier and antagonise CXCL1 signaling in the brain could be a potential therapeutic avenue for HEVA71-associated neurological deficits. Study approval All animal procedures were performed in accordance with the Principles of Laboratory Animal Care and the ethical oversight was approved by the Institutional Animal Care and Use Committee of the National University of Singapore (IACUC-approved number: R20-14766). Patient study was approved by and carried out under the guidelines of the Ethics Committee of the SingHealth Centralised Institutional Review Board (CIRB; CIRB reference number(s): 2012/448/E and H-20-030) under National University of Singapore. Study design We aimed to establish a representative cell model of HEVA71 that closely mimics brain physiology so as to gain a deeper understanding of the mechanisms in HEVA71 neuropathogenesis. We established that cultured primary rat neurons and astrocytes closely recapitulate the key features of HEVA71 infection, thereby establishing its usefulness as an appropriate cell line for modeling HEVA71 neuropathogenesis. We then elucidated the cytokine profiles of HEVA71-infected neuronal cultures so as to identify highly elevated cytokines. Highly elevated CXCL1 in vitro was also detected in CSF of in vivo models and severe HFMD patients; and was subjected to pre-treatment studies in HEVA71-infected neuronal cultures, in which subsequent downstream studies such as protein and viral quantification studies were carried out. We next investigated and affirmed the mechanistic action of CXCL1 in neuronal cultures via protein studies involving lentiviral CRISPR-Cas9 CXCR2 abrogation and ERK1/2 suppression with small molecules. Downstream lentiviral studies involving expression of individual HEVA71 structural and non-structural proteins were performed in neuronal cultures to discover relevant viral protein(s) that induce CXCL1 secretion and/or manipulate CXCR2 signaling cascade in order to trigger HEVA71 neuropathogenesis mechanisms. Further mutation studies were carried out in relevant viral protein(s) to understand how they regulate CXCR2 signaling in vitro and in vivo. All data was collected from 3 independent experiments consisting of triplicates. Cell lines and virus strains Human RD (CCL-136, ATCC) and HEK-293 cells (CRL-1573, ATCC) were maintained in Dulbecco’s Modified Eagle’s Medium (DMEM; Sigma-Aldrich) supplemented with 10% fetal calf serum (FCS; PAA) and 2 g of sodium hydrogen carbonate. HEVA71 strain 41 (Accession no. AF316321.2), HEVA71 strain C2 (Accession no. FJI72159), Coxsackievirus A6 (Accession no. KC866983.1) and Coxsackievirus A16 (Accession no. U05876) were utilized in this study. HEVA71, CA6 and CA16 viruses were propagated in RD cells with DMEM with 2% FCS. UV-inactivated HEVA71 (UI) was prepared via exposure of HEVA71 strains, CA6 or CA16 to ultraviolet light irradiation for 2 h. All live cell culture experiments were carried out in a humidified incubator (37 °C and 5% CO 2 ). Primary neurons and astrocyte cell culture Adult female rats (MPF HanTAc: WH, Wistar) with their corresponding litters (sex undetermined, 8 to 10 pups per time) were purchased from the Centre for Animal resources and housed in temperature controlled (23 ± 1 °C), individually ventilated cages on a 12/12-hour light/dark cycle (7 am to 7 pm) with access to food and water. Primary rat hippocampal neurons or astrocytes were isolated from postnatal day 0 rat pups. Dissected cortices or hippocampi were trypsinized for 30 min prior to addition of serum medium consisting of Modified Eagle’s Medium (MEM; Sigma-Aldrich) supplemented with 5% FCS, 2 mM l -alanyl- l -glutamine (Millipore), 1 x MEM Vitamine (Sigma-Aldrich), Mito+Serum extender (Corning Costar) and 3.8 g/L d -glucose to stop digestion. Digested tissues were triturated with a fire-polished Pasteur pipette and passed through a 40 µm cell strainer (Corning Costar) to remove cell debris. Resulting solution was subjected to centrifugation (500 x g) for 5 min at 25 °C to obtain a clean cell pellet that was resuspended in serum medium. Hippocampal neurons were plated directly on poly-D lysine (PDL; Sigma-Aldrich) coated coverslips in 12-well plates (35,000 cells/well) or PDL-coated 96-well plates (7,000 cells/well) or T-25 culture flasks (100,000 cells/flask) in neuronal plating DMEM/F12 medium (Sigma-Aldrich) and 1 x B27 (Invitrogen). Medium was changed to fresh plating media supplemented with 1 x FUDR (Sigma-Aldrich) after 3 days. Astrocytes were plated on PDL-coated coverslips in 12-well plates (35,000 cells/well) or PDL-coated 96-well plates (7,000 cells/well) in astrocyte plating media (DMEM with 10% FCS). Animal studies All animal work was carried out in accordance with the IACUC-approved protocol (R20-14766) and in Animal Biosafety Level 2 (ABSL2) facility. Adult female mice (BALB/c/CAnNTac) with their corresponding litters (sex undetermined) were purchased from the Centre for Animal resources and housed in temperature controlled (23 ± 1 °C), individually ventilated cages on a 12/12-hour light/dark cycle (7 am to 7 pm) with access to food and water. 1-day-old BALB/c suckling mice (sex undetermined; 26 per group) (Invivos) were infected intracranially with HEVA71 S41 strain or UI or VP4-mutant HEVA71 (2 ×10 7 PFU per mouse) and survival rates and clinical manifestations were monitored for 15 days post infection (dpi) as previously described [38] . For AZD5069 studies, AZD5069 (10 mg/kg) or phosphate-buffered saline (PBS) was administered intracranially at 0, 2 and 4 dpi or intravenously at 0, 2, 4 and 6 dpi following UI or S41 infection in mice (sex undetermined; 25 per group) and monitored for 15 days post infection for survival rates and clinical manifestations. For intracranial Ly6G neutralization studies, IgG isotype (TNP6A7) or anti-Ly6G antibody (BP0075-1) was purchased from BioXcell and administered intracranially at a dose of 1 mg/kg daily from 0 to 5 dpi after UI or S41 infection in mice (sex undetermined; 25 per group). These mice were then monitored for their clinical scores and survival rates till 8 dpi. Severity of clinical symptoms in infected mice were scored by a mice clinical scoring system (Supplementary Table 3 ). Cerebrospinal fluids or sera were collected daily from 0 to 7 or 15 dpi from surviving mice of all groups and quantified for levels of CXCL1 (sex undetermined; 10 per group). Mice brains were harvested from 0 to 15 dpi for subsequent quantification of viral load via plaque reduction assays or for immunohistochemistry and immunoassays. Immunohistochemistry To examine neuropathology and expression of viral antigens and CXCL1, brains from both groups were harvested at 3 to 6 dpi (if mice died at early timepoints due to S41 infection) and 7 dpi (if alive) and fixed with 4% paraformaldehyde (PFA) for 1 week at 4 °C. Sectioning of 80 µm thick free floating coronal sections through the prefrontal cortex and hippocampus were performed using a vibratome (VR1200S, Leica). Sections were collected in cold PBS. Three consecutive sections through each region of interest were alternately stained using Nissl staining or with respective antigen-specific antibodies. Nissl staining was used to evaluate neuronal cell death. Respective sections were mounted on gelatin-coated slides and dried at room temperature. Following treatments with 0.5% crystal violet solution (Sigma-Aldrich), sections were rehydrated in increasing serial concentrations of ethanol and xylene. As a final step, coverslips were applied to the sections. Sections were then digitized at a resolution of 1280 ×960 pixels under a Nikon Eclipse Ci microscope equipped with DS-F12 camera using the NIS Elements software version 5.21.00. To examine the presence of viral antigens, respective sections were treated with 0.3% hydrogen peroxide (Sigma-Aldrich) to remove endogenous catalase activity. After blocking in 3% bovine serum albumin (BSA, Sigma-Aldrich), sections were incubated with mouse anti-HEVA71 antibody (1:200, Millipore, MAB979, clone 422-8D-4C-4D) prior to another overnight incubation with biotinylated anti-mouse secondary antibody (1:400, Santa Cruz, sc2031) at 4 °C. Antibodies used were diluted in BSA. Immunolabelling was developed using the horse radish peroxidase (HRP) conjugated avidin-biotin kit (Vectastain, Vector laboratories) with 0.1% diaminobenzidine as a chromogen. Sections were dried at room temperature on gelatin-coated slides and treated with increasing doses of ethanol and xylene before coverslips were applied. Sections were visualized under a Nikon Eclipse Ci microscope attached with DS-F12 camera through the NIS Elements software. To examine the expression of CXCL1 in neurons, astrocytes and microglia, respective sections were similarly blocked in 3% BSA and incubated with respective combinations of rabbit CXCL1 antibody (1:200, Invitrogen, PA5-86508) and mouse anti-GFAP antibody (1:200, Synaptic Systems, 173011, clone 134B1) with either guinea pig anti-NeuN antibody (1:200, Synaptic Systems, 266004) or guinea pig anti-IBA1 antibody (1:100, Synaptic Systems, 234004). Further overnight incubation was performed with secondary antibodies against mouse Cy2 (715-225-151), Cy3 (715-165-151) or Cy5 (715-175-151), guinea pig Cy2 (706-225-148), Cy3 (706-165-148) or Cy5 (706-175-148), and rabbit Cy2 (711-225-152), Cy3 (711-165-152) or Cy5 (711-175-152) (all dilutions at 1:400, Jackson ImmunoResearch). Sections were dried at room temperature on gelatin-coated slides and treated with increasing doses of ethanol and xylene before coverslips were applied. Sections were visualized using a Zeiss Axio Observer Z1 Microscope equipped with a motorized stage and analyzed via Zeiss Zen 3.4. Study subjects This study was approved by and carried out under the guidelines of the Ethics Committee of the SingHealth Centralised Institutional Review Board (CIRB; CIRB reference number(s): 2012/448/E and H-20-030) under National University of Singapore. Sera samples of healthy and mild HFMD-infected patients were collected from KK Women’s and Children’s hospital with approval from Medical Ethics Committee (reference number: 872.7). CSF samples of moderate HFMD, severe HFMD and other viral encephalitic cases were kindly provided by a clinician (Dr. Ooi Mong How) from their archive that were collected from late 1990 to early 2000, when CIRB or Medical Research and Ethics Committee (MREC) of Ministry of Health (MOH) in Malaysia was not yet established. Diagnosis of patients were evaluated by clinician using clinical case of definition(s) (Supplementary Fig. 10 ). 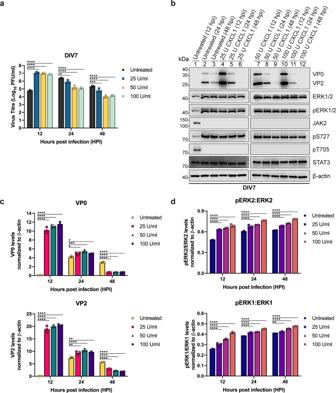Fig. 4: CXCL1 signaling activates     downstream ERK1/2 via CXCR2 to enhance viral replication in     neuronal cultures. aHEVA71 viral titers increase in     CXCL1-pretreated DIV7 neuronal cultures. ExactPvalues for: 25 U/ml at 24 hpi =     0.0033 and 48 hpi = 0.0009.bImmunoblotting of cell lysates from CXCL1-pretreated or     untreated S41-infected DIV7 neuronal cultures against VP0, VP2,     ERK1/2, pERK1/2, JAK2, pS727 (STAT3), pT705 (STAT3) and STAT3.     CXCL1 pre-treatment accelerates the appearance HEVA71 viral     proteins. Elevated pERK1/2 and ERK1/2 levels also emerged     earlier. Immunoblot representative of 3 biological repeats is     shown. Bar charts below show the quantifications for each     protein.cHigh levels of VP0     and VP2 were detectable at 12 hpi only with exposure to CXCL1.     ExactPvalues for VP0: 25     U/ml at 24 hpi = 0.0195, 50 U/ml at 24 hpi = 0.0001 and 100 U/ml     at 24 hpi = 0.002. ExactPvalues for VP2: 25 U/ml at 24 hpi = 0.001 and 100 U/ml at 24 hpi     = 0.0215.dpERK1/2 to ERK1/2     ratios were higher in pretreated cultures versus controls in a     CXCL1 dose-dependent manner at all timepoints. ExactPvalue for pERK1 to ERK1 ratio: 25     U/ml at 48 hpi = 0.0094. β-actin was used as a loading control     for immunoblotting experiments. MOI of 1 was used for all     experiments. Data are expressed as the average with error bars     representing ±SD from 3 independent experiments (n= 3). Statistical analyses were     performed with two-way ANOVA corrected using Bonferroni     post-test. (*P< 0.05, **P< 0.01, ***P< 0.001 and ****P< 0.0001). Source data     are provided as a Source Data file. Sex, number, age of participants and suspected etiologies per group is summarized in Supplementary Table 4 . Clinically-defined HFMD and other viral cases were confirmed using one of the laboratory tests, including viral genotyping and HEVA71, CA6, CA16 or JEV IgM antibody detection. Informed consent was obtained from the parents/guardians of all the recruited subjects from KK Women’s and Children’s hospital to use the sera samples collected. For CSF samples, only verbal consent was obtained. No compensation for participation was provided. Resultant CSF and sera samples were subjected to CXCL1 cytokine measurements. Virus infection studies Neuronal cultures, astrocytes and RD cells were infected with either HEVA71 S41 or HEVA71 C2 strain at MOI of 1, 10 and 50. CA6 and CA16 were used at MOI of 1 to infect neuronal cultures. After incubation with the viruses for an hour, the cell monolayers were washed with phosphate buffered saline (PBS) twice prior to further incubations in virus propagation media. At various time points post-infection, respective cells or supernatants were harvested and processed for cell viability assays, apoptosis assays, plaque assays, immunoblot analyses, quantitative real-time PCR assays, immunofluorescence assays and cytokine analyses. HEVA71 VP4 mutagenesis A glycine (G G C) to alanine (G C C) mutation was carried out at the 5 th position of VP4 gene region in the HEVA71 infectious clone. Part of the HEVA71 infectious clone excluding VP4 genes was amplified by PCR with the appropriate primers using Q5® High-Fidelity master mix protocol. Primers used were purchased from Integrated DNA Technologies (IDT): HEVA71 forward (5’-TCTCCATCCGCTGAG-3’) and reverse (5’-GTTTGATTGTATTGAGGGTTAAT-3’). Subsequently, VP4 gene of HEVA71 infectious clone was mutated and amplified with pair of VP4-mut primers (IDT): VP4-mut forward (5’- TCAATACAATCAAACATGG C CTCACAGGTGTCT-3’) and reverse (5’- CTCAGCGGATGGAGACTTCAGTGGTGCAGCCAT-3’). Of note, the forward primer contained the intended mutation. After agarose gel extraction and purification, both fragments were fused with the In-Fusion® HD cloning kit according to manufacturer recommendations. Generated VP4-mut HEVA71 infectious clone was verified via automated sequencing by Bio Basic Asia Pacific Ltd (Singapore) before upscaling and usage to produce infectious mutant viral particles. VP4-mutant HEVA71 infection studies DIV7 neuronal cultures and RD cells were infected with VP4-mutant HEVA71 at MOI of 1 for an hour. Infected cell monolayers were washed with PBS twice and incubated in virus propagation media. At various time points post-infection, cells or media supernatants were harvested and processed for plaque assays, immunoblot analyses, quantitative real-time PCR assays and cytokine analyses. Cell viability assays Cytotoxicity profiling was carried out in 96-well transparent plates with alamarBlue (Invitrogen) cell viability reagent. Each well consisting of respective cells was washed with PBS twice before the addition of 100 µl of alamarBlue mixture (10 µl of alamarBlue and 90 µl of DMEM with 2% FCS). Following 2 to 4 h of incubation in dark conditions, corresponding fluorescence was measured at excitation wavelength of 560 nm and emission wavelength of 590 nm in TECAN Reader (Infinite 200 PRO series). Respective values were converted to cell viability percentages in comparison to uninfected cells. Apoptosis assays Following various time points (24 or 48 hpi) after HEVA71 infections (S41, C2 or UI) in DIV7 neuronal cultures, respective cells were fixed with 3.7% paraformaldehyde (PFA) prior to TUNEL assays or immunostainings with caspase 3 antibody. For TUNEL assays, the TiterTACs TM Colorimetric Apoptosis Detection Kit (Trevigen) was utilized according to manufacturer’s instructions. Corresponding fluorescence was measured at absorbance wavelength of 450 nm. TAC nuclease and uninfected cells were utilized as a positive and negative control, respectively. For caspase 3 immunostainings, staurosporine (1 uM) and uninfected cells were used as corresponding positive and negative controls. Viral plaque reduction assays A day prior to performing plaque assays, RD cells were seeded in 24-well plates (50,000 to 100,000 cells/well). Cell supernatants or homogenized animal brain tissues from various infection studies were serially diluted 10-fold, ranging from 10 −1 to 10 −7 in DMEM with 2% FCS. Respective diluted solutions were incubated with RD cells from 1 to 1.5 h to allow for viral adsorption. Plates were then washed two times with PBS and added with overlay media of DMEM with 2% FCS and 1% carboxymethylcellulose (CMC). After a 4-day incubation period, cells were fixed and stained with 10% PFA supplemented with 1% crystal violet (Sigma-Aldrich) solution overnight at 25 °C. Mean plaque numbers were counted via visualizing clear patches in respective cell monolayers, which were represented as plaque forming units per milliliter (PFU/ml). Cell extract preparations and immunoblot analyses Cell extracts were prepared with 4 x NuPAGE LDS Sample Buffer (Thermo Fisher Scientific). Quantification of respective cell lysates were performed via Pierce Protein Assay Reagent (Thermo Fisher Scientific) at a wavelength of 660 nm. 10 µg of protein samples were resolved by SDS-PAGE and transferred to nitrocellulose membranes (Bio-Rad) via the Trans-Blot Turbo Transfer System (Bio-Rad). Membranes were blocked with blocking buffer consisting of 5% skim milk (FairPrice) in TBST (150 mM Tris-HCl, pH 7.4, 1.5 M NaCl, 0.5% Tween 20) for 30 min at 25 °C. Membranes were incubated with primary antibodies diluted with blocking buffer overnight at 4 °C. Following three 5-minute TBST washes, membranes were incubated with secondary antibodies. Protein bands were visualized with an enhanced chemiluminescent substrate (Thermo Fisher Scientific) using the C-DiGit Chemiluminescence Western Blot Scanner (LI-COR). Densitometric quantification was performed using ImageJ v1.48 freeware. Band intensities were normalized to actin. The following primary antibodies were used for immunoblotting: mouse anti-HEVA71 antibody (1:2500, Millipore, MAB979, clone 422-8D-4C-4D), mouse anti-actin antibody (1:5000, Millipore, MAB1501, clone C4), rabbit anti-ERK1/2 antibody (1:1000, Cell Signaling Technology, 4695 S), rabbit anti-pERK1/2 antibody (1:1000, Cell Signaling Technology, 4370 S), rabbit anti-pS727 antibody (1:1000, Cell Signaling Technology, 9134 S), rabbit anti-JAK2 antibody (1:1000, Cell Signaling Technology, 3230 S), mouse anti-pT705 antibody (1:1000, Cell Signaling Technology, 4113 S, clone M9C6), mouse anti-STAT3 antibody (1:1000, Cell Signaling Technology, 9139 S, clone 124H6), rabbit anti-CXCR2 antibody (1:1000, Bioss Antibodies, bs1629R), rabbit anti-EGFP antibody (1:5000, Synaptic Systems, 132002), rabbit anti-caspase 3 antibody (1:1000, Cell Signaling Technology, 9662 S), rabbit anti-VP4 antibody (1:5000, Santa Cruz, sc10112W), rabbit anti-V5 antibody (1:1000, Abcam, ab95038) and rabbit anti-pan myristoylation antibody (1:5000, St John’s Laboratory, STJ98665). Secondary antibodies include goat anti-mouse (Bio Rad, 1706516) or rabbit (Bio-Rad, 1706515) IgG (H + L) antibody conjugated with horseradish peroxidase (1:4000, HRP, Bio-Rad). Quantitative real-time PCR (qRT-PCR) assays Following infection, RNA was extracted using the Total RNeasy kit (Qiagen) and treated with DNAse (Promega). qRT-PCR was performed with the StepOne Plus Real-time PCR system (Applied Biosystems). RNA amplification was performed using SYBR green-based RT-PCR kit (Maxima, Thermo Scientific). Primers targeting the 5’ UTR of HEVA71 were: MD90 (5’-ATTGTCACCATAAGCAGCCA-3’) and MD91 (5’-CCTCCGGCCCCTGAATGCGGCTAAT-3’). Resultant values were normalized to actin mRNA , which was quantified using the forward primer (5’-AGCGCGGCTACAGCTTCA-3’) and reverse primer (5’-GGCGACGTAGCACAGCTTCT-3’). All primers were purchased from IDT. Immunoflourescence assays Cells were fixed with 3.7% PFA, and permeablised using 0.3% Triton-X100 (Sigma-Aldrich). After blocking with 10% normal goat serum (NGS; Millipore), cells were incubated with their respective primary antibody combinations for 1 h at 25 °C. After three 10-minute washes in PBS, coverslips were incubated with secondary antibodies for another hour at 25 °C and washed again thrice with three PBS washes with 10-minute intervals. As a final step, coverslips were mounted with Fluoro-Gel II with DAPI (Electron Microscopy Sciences) on glass slides and visualized using a Zeiss Axio Observer Z1 Microscope equipped with a motorised stage. Images were analyzed on Zeiss Zen 3.4. The following primary antibodies were utilized for immunostainings: mouse anti- dsRNA antibody (1:500, Merck, MABE1134, clone rJ2), guinea pig anti-Tau antibody (1:400, Synaptic Systems, 314004), rabbit anti-GFAP antibody (1:1000, Synaptic Systems, 173002), mouse anti-GFAP antibody (1:500, Synaptic Systems, 173011, clone 134B1), guinea pig anti-NeuN antibody (1:400, Synaptic Systems, 266004), mouse MAP2 (1:1000, Sigma-Aldrich, M4403, clone HM-2), rabbit caspase 3 antibody (1:1000, Cell Signaling Technology, 9662 S) and goat CXCL1 antibody (1:200, Invitrogen, PA546932). Secondary antibodies against mouse Cy2 (715-225-151), Cy3 (715-165-151) or Cy5 (715-175-151), guinea pig Cy2 (706-225-148), Cy3 (706-165-148) or Cy5 (706-175-148), goat Cy2 (705-225-147), Cy3 (705-165-147) or Cy5 (705-175-147) and rabbit Cy2 (711-225-152), Cy3 (711-165-152) or Cy5 (711-175-152) was used (1:400, Jackson ImmunoResearch). Cytokine analyses Culture supernatants from HEVA71-infected neurons, HEVA71-infected astrocytes and lentiviral-infected neurons or CSF and sera taken from mice or human clinical cases over various time/day points were assayed using the respective Bio-Plex Pro rat cytokine 23-plex kit (Bio-Rad) or rat CXCL1 ELISA kit (Aviva Systems Biology) or human CXCL1 ELISA kit (ThermoFisher Scientific) according to manufacturer’s instructions. Data from the Bio-Plex assays were processed using Bio-Plex Manager software version 6.1 (Bio-Rad). Cytokines with out-of-range readings that were below its detection limits were recorded as 0.1 pg/ml. Compound preparations Recombinant rat CXCL1 (25 µg) was purchased from Peprotech and diluted in water to yield 100,000 U/ml stock solution. FR180204 (5-(2-phenylpyrazolo[1,5-a]pyridin-3-yl)−1 H -pyrazolo[3,4-c]pyridazin-3-amine) was obtained from Sigma-Aldrich and diluted in water to obtain a 10 mM stock solution. AZD5069 (10 mg) was purchased from MedChem Express and diluted in PBS to achieve a 25 mM stock solution. Stock solutions were stored at −20 °C. Compound treatment assays Cultures were pretreated with a range of CXCL1 concentrations (0 to 100 U/ml) for 24 h prior to HEVA71 S41 infection at MOI of 1. Supernatants of DIV7 neuronal cultures were collected at 12, 24 and 48 hpi and plaque reduction assays were performed for viral titer quantifications. Lysates from DIV7 neuronal cultures were also harvested and subjected to immunoblot analyses. DIV7 neuronal cells were separately seeded in 96-well plates and treated with a range of doses of FR180204 (1.25 to 20 µM) or AZD5069 (0 to 750 nM) for 48 h, before relevant cell viabilities for each dosage were measured via cell viability assays. Following 100 U/ml of CXCL1 pre-treatments of DIV7 neurons, cells were infected with HEVA71 (S41) for an hour. After washing twice with PBS, 5 µM of FR180204 or 750 nM of AZD5069 was added in fresh neuronal culture maintenance media to HEVA71-infected neurons, where cells were further incubated for 12, 24 and 48 h prior to cell lysis and subsequent immunoblotting assays. CRISPR-Cas9 deletion of CXCR2 The following sgRNA against CXCR2 were designed using sgRNA Designer (Broad Institute), (5’-GCTGTCAGGGCTGGTTGAAC-3’, 5’-CTCAAGGCTTGGGAGCTGTC-3’, 5’- GGCTTGGGAGCTGTCAGGGC-3’). The resultant oligonucleotides were purchased from IDT, and inserted into LentiCRISPRv2 plasmid (Addgene, plasmid #52961, a kind gift from Dr. Feng Zhang) at the BsmBI restriction enzyme site. sgRNA lentiviruses were produced by co-transfecting individual pLenti-CRISPR- CXCR2 -sgRNA vectors with pMDL/pRRE, pRSV-rev and pMD2.G helper plasmids in DMEM supplemented with 3% FCS for lentiviral production and purified as previously described [87] . Lentiviruses expressing LUC sgRNA (5’-TCATATTCGTTAAAGCCCGG-3’) were employed as controls. 6 days following infection with control or CXCR2- sgRNA expressing lentiviruses, DIV7 neuronal cultures were pre-treated with 100 U/ml of CXCL1 prior to HEVA71 infection at MOI of 1 and subjected to downstream immunoblot assays. Lentiviral transduction of HEVA71 proteins Individual HEVA71 proteins were separately expressed in DIV7 neuronal cultures. Specifically, cDNAs encoding full-length HEVA71 (S41) VP1, VP2, VP3, VP4, VP4-mut, 2 A, 2B, 2 C, 3 A, 3B, 3 C or 3D were separately cloned into the FHUG-EGFP backbone (Addgene, plasmid #14883, a kind gift from Dr. David Baltimore) using the EcoRI and AgeI sites. 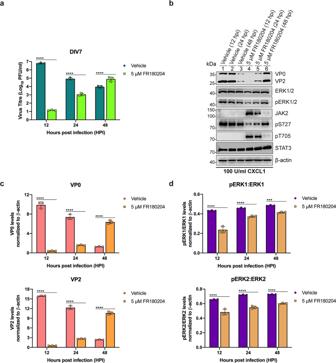Fig. 5: Blocking CXCL1 signaling     by pERK1/2 inhibition reduces viral replication in neuronal     cultures. aInhibiting ERK1/2 decreased viral titers at 12     and 24 hpi in DIV7 neuronal cultures.bImmunoblotting of S41-infected DIV7 neuronal     cultures treated simultaneously with FR180204 (5 µM) and CXCL1     (100 U/ml) at 12, 24 and 48 hpi. ERK1/2 inhibition delays the     expression of HEVA71 viral proteins. Immunoblot representative     of 3 biological repeats is shown. Bar charts below show the     quantifications for each protein.cVP0 and VP2 levels decreased at 12 and 24 hpi     with ERK1/2 inhibition.dpERK1/2 to ERK1/2 ratios were reduced at all timepoints in     FR180204-treated cultures. ExactPvalue for pERK1 to ERK1 ratio with FR180204 at     48 hpi = 0.0001. β-actin was used as a loading control for     immunoblotting experiments. MOI of 1 was used for all     experiments. Data are expressed as the average with error bars     representing ±SD from 3 independent experiments (n = 3).     Statistical analyses were performed with two-way ANOVA corrected     using Bonferroni post-test. (***P< 0.001 and ****P< 0.0001). Source data     are provided as a Source Data file. Primers (IDT) used are indicated in Supplementary Table 5 . The P2A cleavage sequence was inserted between the viral proteins and EGFP. Following their expression, the EGFP moiety is cleaved to allow for the expression of native viral proteins. VP4-mut cDNA was obtained via a site-directed mutagenesis (MGXXXS to MAXXXS) with In-Fusion Cloning kit (Takara) according to manufacturer’s instructions (Supplementary Table 5 ). Empty FHUG-EGFP plasmid was utilized as EGFP expression control. Production of individual lentiviruses with each HEVA71 protein were performed as mentioned above and stored in 100 µl aliquots at −80 °C until use. Neuronal cultures were fixed for immunofluorescence staining or lysed for immunoblotting at 6 days after lentiviral infection. Culture supernatants were also collected and subjected to CXCL1 cytokine analyses. Immunoprecipitation assays Using In-Fusion Cloning kit (Takara), a V5 tag was introduced from pcDNA3.1/nV5-DEST vector (Addgene, plasmid #12290010) into FHUG-EGFP-VP4 and FHUG-EGFP-VP4-mut according to manufacturer’s instructions. 200 µl of concentrated lentiviruses expressing VP4 or VP4-mut tagged with V5 were then used to infect DIV1 neurons seeded in T-25 flasks. Empty FHUG-V5 plasmid was used as a control. After 6 days post infection, cells were washed with PBS twice and lysed with 500 µl of HEPES Lysis Buffer TBST (50 mM HEPES, 150 mM NaCl, 1 mM EDTA, 1% Triton-X100, pH 7.2) supplemented with protease inhibitor cocktail (100X; Thermo Fisher Scientific). Lysates were clarified by centrifugation at 10,000 g for 10 min at 4 °C. Resultant supernatants were collected and added with 1 µl of anti-V5 antibody (1:200, Abcam, ab95038) for subsequent incubations at 4 °C for 3 to 4 h. 30 µl of agarose beads (Thermo Fisher Scientific) were then washed three to five times with HEPES Lysis Buffer and added to each antibody-lysate mixture for another 1 to 2 h of incubation. Following this, resultant mixtures were spun down at 1000 x g at 1 min at 4 °C and supernatants were removed. Beads were washed thrice in HEPES lysis buffer through inverting them 6 times and removing lysis buffer via centrifugation at 12,000 x g for 1 min at 4 °C. Immune complexes were then eluted from beads by adding 2 x NuPAGE LDS Sample Buffer (Thermo Fisher Scientific) and resolved by subsequent SDS-polyacrylamide gel electrophoresis. Proteins were transferred to nitrocellulose membranes (Bio-Rad) and further incubated with appropriate antibodies. Fluorescence-activated cell sorting (FACS) analysis Leukocyte and neutrophil populations for FACS analyses were obtained as described previously [88] , [89] . Brain and muscle tissues from individual animals were separately minced gently in RPMI 1640 medium (Thermo Fisher Scientific) with a razor blade and incubated with collagenase D (Roche; 1 mg/ml) and DNAse I (Roche; 50 µg/ml) for 30 min at 37 °C. Digested tissues were passed through a 70 µm cell strainer (Corning Costar) to remove cell debris and to obtain single cell suspensions. 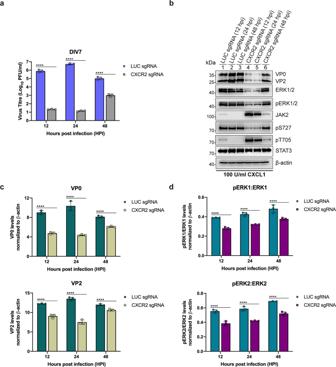Fig. 6: Blocking CXCL1 signaling     by CXCR2 deletion decreases viral replication in neuronal     cultures. aCXCR2deletion in infected neuronal cultures reduced viral titers at     all time points tested.bLysates from neuronal cultures infected with control (LUCsgRNA)-or CXCR2sgRNA-expressing lentiviruses were     similarly immunoblotted as ina.CXCR2deletion     delays viral protein expression in neuronal cultures despite     CXCL1 pretreatment. Immunoblot representative of 3 biological     repeats is shown. Bar charts below show the quantifications for     each protein.cVP0 and VP2     levels decreased at all timepoints inCXCR2-deleted samples.dpERK1/2 to ERK1/2 ratios were decreased inCXCR2-deleted samples.     β-actin was used as a loading control for immunoblotting     experiments. MOI of 1 was used for all experiments. Data are     expressed as the average with error bars representing ±SD from 3     independent experiments (n= 3). Statistical analyses were performed with     two-way ANOVA corrected using Bonferroni post-test.         (****P< 0.0001).     Source data are provided as a Source Data file. Cells were spun down at 500 x g for 5 min at 4 °C. The resultant cell pellets from brain tissues were resuspended in ice-cold 90% Percoll (Sigma Aldrich) and overlaid with 60% Percoll, followed by 40% Percoll and subsequently HBSS (Thermo Fisher Scientific) gently. Cell pellets obtained from muscles were resuspended with 70% Percoll and gently covered with 37% Percoll followed by 30% Percoll. All Percoll solutions were diluted in HBSS. Cells were isolated by centrifugation at 600 x g for 30 min at 4 °C. Braking was not used for deceleration. The cell fraction (containing leukocytes) located between the 60% and 40% interphase (for brains) and 70% and 37% phases (for muscles) were carefully aspirated. HBSS was added to the cell suspensions, which were spun again at 550 x g for 10 min at 4 °C. Resultant cell pellets were resuspended in 100 µl FACS buffer (Sigma Aldrich). Samples were stained with fluorescent isothiocyanate (FITC)-conjugated anti-mouse Ly6G antibody (1:100, BD Biosciences, BD551460), PE-Cy7-conjugated anti-mouse CD45 antibody (1:200, eBioscience, 25-0453-82) and Calcein violet AM (1:200, Invitrogen, C34858) in the dark at 4 °C for 30 min. Cells were then pelleted by centrifugation at 400 x g at 4 °C for 5 min and washed twice with FACS buffer prior to analyses using the FACSCalibur flow cytometer (BD Biosciences). 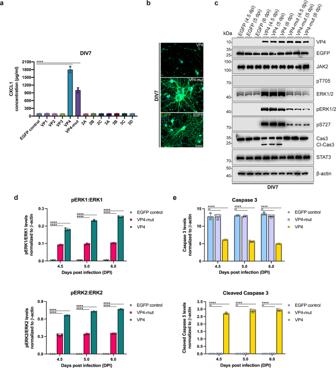Fig.     7: HEVA71 VP4 induces     CXCL1 secretion for HEVA71 replication and subsequent viral     neuropathogenesis in neuronal         cultures. aCXCL1 levels were elevated in culture     supernatants when VP4 and VP4-mut were expressed. Higher levels     of the chemokine were detected in samples expressing wildtype     VP4.bImmunofluorescence     images of control (EGFP)- or VP4 (wildtype and mutant)-     expressing neuronal cultures. Neurite disintegration was only     observed in wildtype VP4-expressing neuronal cultures. Scale     bars represent 20 µm.cImmunoblots of cell lysates from control (EGFP)-, VP4- or     VP4-mut-expressing neurons against VP4, EGFP, ERK1/2, pERK1/2,     pS727 (STAT3), JAK2, pT705 (STAT3), STAT3, caspase 3 and cleaved     caspase 3. Immunoblot representative of 3 biological repeats is     shown. Bar charts below show quantifications for each protein.dpERK1/2 to ERK1/2 ratios     were higher in VP4-expressing neuronal cultures as compared to     VP4-mut or EGFP controls at all time points.eCleaved caspase 3 was detected only     in VP4-expressing neuronal cultures. ExactPvalue for caspase 3: VP4-mut at 6     dpi = 0.6026. β-actin was used as a loading control for     immunoblotting experiments. Data are expressed as the average     with error bars representing ±SD from 3 independent experiments         (n= 3). Statistical     analyses were performed with two-way ANOVA corrected using     Bonferroni post-test. (ns > 0.9999 unless specified, and         ****P< 0.0001).     Source data are provided as a Source Data file. Data collected were analyzed using FlowJo TM version 10.8. Fluorescence-activated cell sorting (FACS) gating strategy Cells of interest were gated on forward scatter area (FSC-A)/side scatter area (SSC-A) plot to remove cell debris. Single cells were subsequently gated on forward scatter height (FSC-H)/forward scatter area (FSC-A) and forward scatter width (FSC-W)/forward scatter area (FSC-A) density plots to exclude doublets. Live leukocytes were identified by selecting cells that are dually positive for Calcein violet AM and CD45. These cells were then further gated for neutrophils that are both CD45- and LY6G- positive. Data were analyzed using FlowJo TM software and population frequencies were expressed as percent of single cell population. Statistical analysis Statistics were performed via GraphPad Prism 9 version 9.3.0. All experiments were performed three independent times with 3 technical replicates. 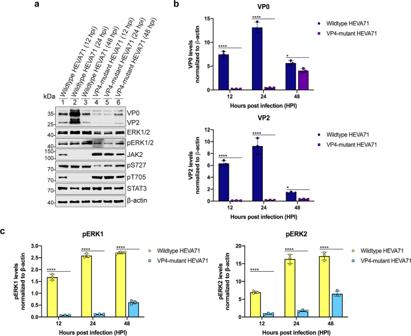Fig.     8: VP4-mutant HEVA71     reduces CXCL1 signaling and subsequent HEVA71 replication in     neuronal cultures. aImmunoblots of cell lysates from wildtype     HEVA71 and VP4-mutant HEVA71-infected DIV7 neuronal cultures at     12, 24 and 48 hpi. Similar primary antibodies excluding caspase     3 were used. VP4 mutation delays the expression of HEVA71 viral     proteins. Immunoblot representative of 3 biological repeats is     shown. Bar charts below show quantifications for each protein.bVP0 and VP2 levels     decreased at all time points in neurons infected with VP4-mutant     HEVA71. ExactPvalues for:     VP0 at 48 hpi = 0.018 and VP2 at 48 hpi = 0.0161.cpERK1/2 levels were decreased in     VP4-mutant HEVA71-infected neurons. Data are expressed as the     average with error bars representing ±SD from 3 independent     experiments (n= 3).     Statistical analyses were performed with two-way ANOVA corrected     using Bonferroni post-test. (*P< 0.05 and ****P< 0.0001). Source data are provided as     a Source Data file. Data are represented as means and standard deviations (SDs), calculated by Microsoft Excel 2016/version 16.56. Two-way ANOVA followed by post hoc test for multiple comparisons was utilized in determining statistical significance, as described in figure legends. p ≤ 0.05 was considered significant. 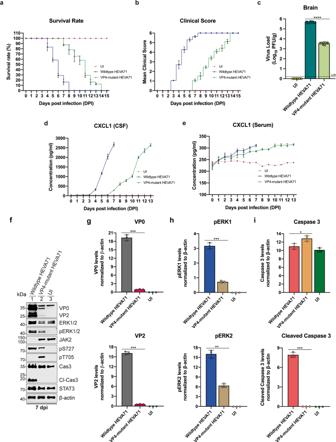Fig.     9: Mutating HEVA71 VP4     reduces CXCL1 signaling and associated HEVA71 replication and     neuropathogenesis in mice. a–eInfection of mice with wildtype or VP4-mutant     HEVA71 virons.aSurvival rates     andbmean clinical scores of     mice infected with wildtype, VP4-mutant or UI virus. Wildtype     and VP4-mutant HEVA71-infected mice displayed mortality and high     clinical scores from 4 and 7 dpi, respectively. UI-infected mice     were healthy till 15 dpi.cVP4-mutant HEVA71-infected mice had lower viral loads detected     in their brains at 7 dpi. UI-infected mice were used as     controls. Negligible viral loads were detected below limit of     detection (LOD = 0.2).d,eCXCL1 levels were highly     elevated indCSF but only     slightly elevated ineserum of     both wildtype and VP4-mutant HEVA71-infected mice but not in     UI-infected mice. Wildtype HEVA71-infected mice showed     increasing CXCL1 from 4 dpi but those for VP4-mutant-infected     mice emerged at 7 dpi.fBrain     lysates of wildtype, VP4-mutant or UI-infected mice were     analyzed by immunoblotting at 7 dpi. Infection with VP4-mutant     HEVA71 delays the expression of HEVA71 viral proteins.     Immunoblot representative of 3 biological repeats is shown. Bar     charts below show quantifications for each protein.gVP0 and VP2 levels decreased at 7     dpi with VP4-mutant HEVA71. ExactPvalues for: VP0 = 0.0009 and VP2 = 0.0002.hpERK1/2 were reduced in     VP4-mutant HEVA71-infected mice. ExactPvalues for: pERK1 = 0.0009 and pERK2 = 0.0012.iCleaved caspase 3 was     detected in wildtype HEVA71-infected mice but not VP4-mutant     HEVA71-infected mice at 7 dpi. ExactPvalues for: caspase 3 = 0.0254 and cleaved     caspase 3 = 0.0008. β-actin was used as a loading control for     immunoblotting experiments. Data are expressed as the average     with error bars representing ±SD from 3 independent experiments         (n= 3). Statistical     analyses were performed with two-way ANOVA corrected using     Bonferroni post-test. (**P< 0.01, ***P< 0.001 and ****P< 0.0001). Source data     are provided as a Source Data file. 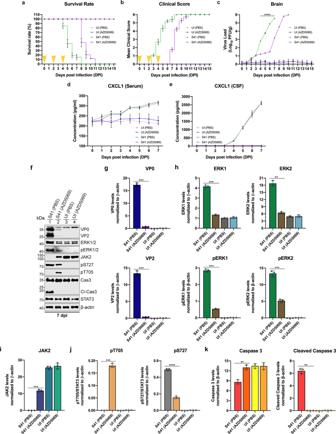Fig.     10: Suppressing CXCL1     signaling by AZD5069 treatment improved survival and clinical     scores that correlated with reduced HEVA71 viral load in     infected mice. aSurvival rates andbmean clinical scores of mice infected with S41     or UI with or without AZD5069 treatment, respectively.     Arrowheads indicate time points of AZD5069 administration.     S41-infected mice displayed mortality and high clinical scores     from 4 dpi. AZD5069 administration to S41-infected mice delayed     mortality and high clinical scores until 8 dpi. UI-infected mice     were healthy till 15 dpi.cAZD5069 treatment lowered viral loads in brains of S41-infected     mice from 4 to 7 dpi.d,eCXCL1 levels were     slightly elevated indserum     but highly elevated ineCSF of     S41-infected mice with or without AZD5069 but not in UI-infected     mice.fBrain lysates of S41-     or UI-infected mice with or without AZD5069 treatment were     subjected to immunoblotting analyses at 7 dpi. AZD5069 treatment     delays the expression of HEVA71 viral proteins. Immunoblot     representative of 3 biological repeats is shown. Bar charts     below show quantifications for each protein.gVP0 and VP2 levels decreased at 7     dpi with AZD5069 treatment. ExactPvalues for: VP0 = 0.0006 and VP2 = 0.0009.hpERK1/2 and ERK1/2 levels     were reduced in AZD5069-treated mice. ExactPvalues for: ERK1 = 0.0002,     ERK2 = 0.0013, pERK1 = 0.0001 and pERK2 = 0.0007.iJAK2 levels persisted in     CXCR2-suppressed mice with S41 infection. ExactPvalues for: JAK2 = 0.001.jAZD5069 treatment     increased phosphorylation of STAT3 at pT705 but decreased pS727     levels at 7 dpi. ExactPvalues for: pT705 = 0.0007.kCleaved caspase 3 was detected only in S41-infected mice without     AZD5069 treatment at 7 dpi. ExactPvalues for: caspase 3 = 0.0013 and cleaved     caspase 3 = 0.0015. β-actin was used as a loading control for     immunoblotting experiments. Data are expressed as the average     with error bars representing ±SD from 3 independent experiments         (n= 3). Statistical     analyses were performed with two-way ANOVA corrected using     Bonferroni post-test. (**P< 0.01, ***P< 0.001 and ****P< 0.0001). Source data     are provided as a Source Data file. N values are also indicated within figure legends and refer to biological replicates, whereas technical replicates (included in Source Data file) refer to repeated analysis of the same samples. Derived statistics correspond to analysis of averaged values across biological replicates, and not pooled technically and biological replicates. Reporting summary Further information on research design is available in the Nature Research Reporting Summary linked to this article.